A 3D insight on the catalytic nanostructuration of few-layer graphene The catalytic cutting of few-layer graphene is nowadays a hot topic in materials research due to its potential applications in the catalysis field and the graphene nanoribbons fabrication. We show here a 3D analysis of the nanostructuration of few-layer graphene by iron-based nanoparticles under hydrogen flow. The nanoparticles located at the edges or attached to the steps on the FLG sheets create trenches and tunnels with orientations, lengths and morphologies defined by the crystallography and the topography of the carbon substrate. The cross-sectional analysis of the 3D volumes highlights the role of the active nanoparticle identity on the trench size and shape, with emphasis on the topographical stability of the basal planes within the resulting trenches and channels, no matter the obstacle encountered. The actual study gives a deep insight on the impact of nanoparticles morphology and support topography on the 3D character of nanostructures built up by catalytic cutting. The arrangement of sp 2 -bonded carbon atoms in a bi-dimensional structure leads to the unique physical, chemical and mechanical properties of single-layer graphene [1] . Among these properties, the high electronic conductivity, good thermal and chemical stability and high surface area promote graphene (single or few-layer) as an ideal material to be used for different applications, as, for instance, a support in the catalysis field for both liquid- and gas-phase reactions [2] . As compared with other types of supports, graphene may participate as well directly as a catalyst after being doped with different elements [3] , [4] , [5] . By strictly adjusting the graphene surface properties [6] , [7] and the number of layers [8] , one gets a close control of the active phase distribution on its surface in terms of size, shape and density, and this has a strong impact on the final properties of the catalytic system. The catalysis field is a gigantic materials consumer and so far the mass production of graphene and few-layer graphene (FLG) remains a challenge. Although several preparation methods of large quantities of FLGs were described up to now, the FLG properties are dominated by the bulk properties of graphite (low density and surface accessibility) [2] . As the graphene sheets have a strong tendency to restack through van der Waals forces on drying, the surface areas are strongly reduced and, therefore, these systems are no longer adapted for catalytic applications, particularly for gas-phase reactions. One strategy advanced for overcoming this drawback is the nano-structuration of FLG sheets by catalytic hydrogenation, which will create highly accessible nano-channels on the FLG surface. These nano-channels will most probably favour the development of new anchorage sites on the FLG surface, where the metallic and/or oxide active phases will adhere. The catalytic hydrogenation of graphite using metals from Group VIII was a process intensively studied in the last decades in the framework of hydrocarbon production from coal [9] , [10] . In principle, when a metal nanoparticle (NP) attached to a carbon-based structure is submitted to a hydrogen flow at high temperature, it starts etching the carbon atoms along well-defined crystallographic axes, generating methane as reaction product. After the discovery of graphene [11] , a significant amount of studies predicted that the graphene properties can be tuned by assembling graphene in one-dimensional structures with different shapes, size and edge configurations, called graphene nanoribbons [12] , [13] , [14] , [15] . They can be synthetized, for instance, by FLG cutting during the catalytic hydrogenation using metal-based NPs. The role of NPs nature (Ni, Co, Fe and Pt), size, structure and initial localization, as well as the importance of the hydrogenation conditions (H 2 pressure and temperature) as criteria controlling the cutting process have been highlighted by different investigations [16] , [17] , [18] , [19] , [20] , [21] , [22] , [23] . Moreover, a recent study has shown the improvement of the adsorption capacity of CO 2 molecules on the catalytically nanostructured FLG as compared with the unstructured FLG [22] . These studies highlight the most important factors influencing the catalytic cutting process and call for a better understanding of the cutting process. So far, a detailed investigation of the phenomenon is missing because most of the studies only use a two-dimensional (2D) approach regardless of the number of the graphene sheets and the interface between the NPs and the graphene’s surface. It is worth mentioning that even with the use of scanning tunnelling microscopy, the ability of resolving in-depth details and to obtain a real three-dimensional (3D) image of the cutting process is still missing. In this general framework, we have recently developed a synthesis method able to produce large amounts of high-quality FLGs through a mechanical ablation of pencil lead [24] , [25] . Iron oxide (Fe 3− x O 4 ) NPs with homogeneous size were first deposited on FLGs and the as-obtained composite has been exposed to a H 2 atmosphere at high temperature for producing new nanostructures. This approach enables one to create geometrical trenches with well-defined depths, widths and crystallographic orientations. To characterize the catalytic cutting process and deeply explore the characteristics of such nanostructure, we used an approach combining electron tomography with high-resolution transmission electron microscopy (HR-TEM) and spatial-resolved electron energy loss spectroscopy (EELS). This work provides original insights on the 3D shape of the etched trenches and their localization in relation to the FLG surface, as correlated with the FLG topographical events: steps and edges. Under controlled conditions, the active NPs create trenches and tunnels with orientations, lengths and morphologies defined by the crystallography and the topography of the carbon substrate. The trench shape is defined by the 3D character of the active NP and its basal plane does not change no matter what topographical features the active NP crosses. Sample preparation The FLG sheets have been synthesized by mechanical ablation of pencil leads assisted by an ultrasonication process. The decoration of the FLG surface by homogeneous Fe 3− x O 4 NPs was carried out using a solvothermal synthesis method [26] , [27] . The etching of FLG sheets was performed at 800 °C in a H 2 atmosphere (see Methods for more details). TEM, HR-TEM and scanning TEM–EELS investigations TEM micrographs of the iron-based NPs dispersed on the FLG support are displayed in Fig. 1 . 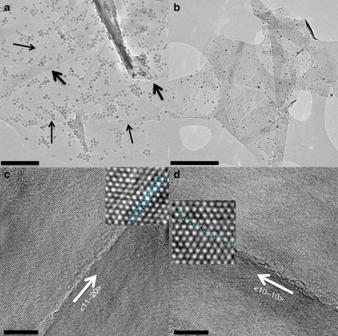Figure 1: Two-dimensional global view and high-resolution imaging of the nanostructured system. TEM images of typical Fe-based NPs onto FLG sheets before (a) (scale bar, 100 nm) and after (b) (scale bar, 200 nm) the catalytic cutting under hydrogen flow. HR-TEM images illustrating the preferential crystallographic orientation of trenches with zigzag (c) and armchair (d) edge morphologies (scale bars 5 nm). Figure 1a presents a TEM image taken from a typical FLG sheet, after deposition of Fe 3− x O 4 NPs only. The analysis of TEM images shows that the morphology of an individual aggregate is dominated by the presence of successive terraces constituted on the FLG surface, due to the superposition of several individual sheets (see thick arrows), whereas several steps can be observed on single FLG sheets (see thin arrows). The NPs have a narrow size distribution, with a mean diameter of ~7±2 nm and a good dispersion on the FLG surface and a preferential localization at the steps. The morphology of the FLG sheets after the hydrogen-assisted treatment is presented in Fig. 1b . As compared with the sample before the catalytic hydrogenation, various types of NPs with sizes ranging from 7 to 100 nm along with different internal structures and geometrical configurations are identified ( Supplementary Fig. 1 ). A detailed spatial-resolved scanning TEM–EELS (STEM–EELS) analysis revealed that the catalytic activity can be associated to both pure metallic iron and iron oxide NPs ( Supplementary Fig. 2 ). However, one cannot exclude that some of the oxide-rich shells have been formed after cutting, once the particles are in contact with air. By considering particularly the NPs with incomplete iron-oxide shell, one can identify the metallic part always in the NP front side. The trenches created by metallic iron appear to be generally longer and better defined as compared with those generated by the iron oxide. No iron carbide phase has been detected. The EELS investigation of the hollow small NPs identified their complete oxidation ( Supplementary Fig. 2b ). Trench lengths are between 30 nm and 1 μm, while their widths stay between 10 and 100 nm. The trenches widths remain constant from the beginning to the end, allowing one to conclude that NPs size does not change significantly during the cutting and no faceting or chemical modification occurred. As a consequence, the difference within the channel widths can be attributed to the various sizes of the NPs as obtained during the temperature increment before the cutting process. The broadening of particle size distribution can be attributed to the NP sintering, which strongly depends on the particle localization while heating. This topic has already been studied for the case of platinum NPs, to a lesser extent [28] . The current HR-TEM analysis ( Fig. 1c,d ) show that the well-defined trenches are not randomly oriented but follow specific crystallographic directions, that is, <11–20> and <10–10> a topic well documented in the literature [16] , [18] , [19] . Figure 1: Two-dimensional global view and high-resolution imaging of the nanostructured system. TEM images of typical Fe-based NPs onto FLG sheets before ( a ) (scale bar, 100 nm) and after ( b ) (scale bar, 200 nm) the catalytic cutting under hydrogen flow. HR-TEM images illustrating the preferential crystallographic orientation of trenches with zigzag ( c ) and armchair ( d ) edge morphologies (scale bars 5 nm). Full size image Electron tomography Based on the electron tomography analysis, we were able to access crucial information on the exact topography of a FLG sheet. The analyses were thus carried out on several region of the catalytically etched system to get a deep understanding on the cutting process. 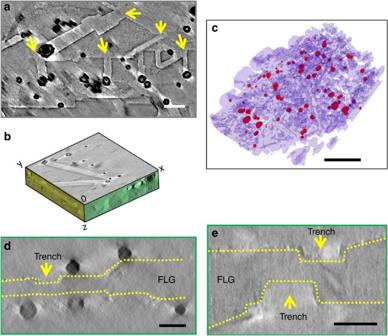Figure 2: Three-dimensional overview of the catalytic cutting process: NPs and trenches. (a) XY slice extracted from the reconstructed volume of a nanostructured FLG area (scale bar, 20 nm). Yellow arrows point to the initial position of the active NPs. (b) 3D representation of the specimen reconstruction: XY plane in grey, XZ in green and YZ in yellow. (c) 3D model displaying a general view of the analysed fragment. NPs are presented in red, whereas the mauve colour indicates the FLG sheet (scale bar, 500 nm). XZ slices extracted from the reconstructed volumes showing NPs (d) and trenches (e) on both sides of the FLG sheets (scale bars, 20 nm). Figure 2a for instance depicts a longitudinal slice (perpendicular to the incident electron beam at 0° tilt). All the active NPs, that is, those participating to the cutting process, are those located initially at the edges of the pristine FLG or at the steps, whereas the NPs situated on the FLG flat surface appear to be generally inactive. Accordingly, one may state that the driving force responsible for cutting closely relates to the interaction between NPs and carbon atoms of the support localized on the edge of the terrace. The contact between the front side of the NP and the carbon atoms from an edge or a step creates a higher interaction than the one between the carbon basal plane and the bottom side of the NP [9] , [23] . A sketch in Fig. 2b presents the xyz orientations of the slices from the reconstructed volumes in the geometrical configuration that will be further employed in the current report. Figure 2c displays a model of NPs distribution on the FLG support obtained using the discrete algebraic reconstruction technique (DART) algorithm. By analysing the simultaneous iterative reconstruction technique (SIRT) reconstructed volume slice by slice in cross-section, one identifies NPs on both sides of the FLG support ( Fig. 2d ). It is important to mention that the localization of iron-based NPs on both sides of the FLG has no impact on the cutting process, as trenches have been created on both sides of the support (see Fig. 2e ). According to the cross-section views presented, the trench walls are not perfectly straight in terms of their atomic arrangement especially for the ‘open-surface’ trenches. However, note that the tomographic resolution achieved in our reconstruction is about 1 nm in the z direction and, therefore, our hypothesis should be delimited accordingly. For a clearer view of the NPs distribution relative to the FLG sheet, see the Supplementary Movie 1 . Figure 2: Three-dimensional overview of the catalytic cutting process: NPs and trenches. ( a ) XY slice extracted from the reconstructed volume of a nanostructured FLG area (scale bar, 20 nm). Yellow arrows point to the initial position of the active NPs. ( b ) 3D representation of the specimen reconstruction: XY plane in grey, XZ in green and YZ in yellow. ( c ) 3D model displaying a general view of the analysed fragment. NPs are presented in red, whereas the mauve colour indicates the FLG sheet (scale bar, 500 nm). XZ slices extracted from the reconstructed volumes showing NPs ( d ) and trenches ( e ) on both sides of the FLG sheets (scale bars, 20 nm). Full size image To highlight the one-to-one correspondence between the trenches and the associated NPs we have analysed cross-sections within the volume, by focusing on NPs and the FLG topography within the very same trench ( Fig. 3a ). At this stage of analysis one might assume that the main factor imposing the trench profile is the 3D character (shape and morphology) of the active NPs. By superimposing the cross-section analyses within the trench profile (yellow line) close to its end with the NPs profile (white line) from the end of its trajectory ( Fig. 3b ), one identifies a close correspondence between the trench width and the section of the NP contacting the channel border. Note that the superposition is not perfect at the atomic level. To explain this, let us notice that the trench width can slightly vary along its length, as the NPs size and shape might change in the trench longitudinal direction due to the continuous restructuring of the particle surface during cutting. At this extent, a schematic representation of the cutting process can be associated to the relation between the initial NPs position and their activity, see Fig. 3c . Another finding evidenced by this representation relates to the FLG atomic roughness as well as the non-regular shape of the cutting particle. An explanation for these particular morphologies can be searched by following two directions: first, the FLG preparation method is susceptible to provoke atomically non-flat supports, and second the complex hydrogenation reaction taking place at the surface of the particle would most probably alter its initially regular shape. 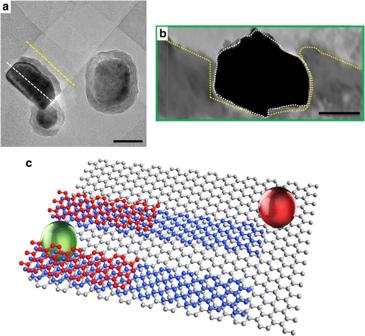Figure 3: The relationship between the active NP and the corresponding trench. (a) TEM projection of a trench and the corresponding digging NP (scale bar, 20 nm). (b) Superposition of the XZ slices of the NP (white line inFig. 3a) and the trench (yellow line) showing the close relationship between the 3D shape of the NP and the trench profile created (scale bar, 10 nm). (c) Schematic illustration of the crystallographic cutting of an FLG sheet by iron-based NPs sitting at different locations (on the planar surface (red) and at the steps (green)). Figure 3: The relationship between the active NP and the corresponding trench. ( a ) TEM projection of a trench and the corresponding digging NP (scale bar, 20 nm). ( b ) Superposition of the XZ slices of the NP (white line in Fig. 3a ) and the trench (yellow line) showing the close relationship between the 3D shape of the NP and the trench profile created (scale bar, 10 nm). ( c ) Schematic illustration of the crystallographic cutting of an FLG sheet by iron-based NPs sitting at different locations (on the planar surface (red) and at the steps (green)). Full size image By applying the same approach to other pairs of trench/NP, we were able to analyse the 3D shape changes of the trench along its length as function of the topography of the FLG along the cutting length, that is, constant and variable thickness. In the case of a constant thickness of the FLG support, the analysis of individual trenches shows that their depths are constant during cutting, as shown in Supplementary Fig. 3 . In this case, the NP uses about one-third of its diameter (~6 nm) for cutting and this correspond to the trench depth. The height of the step where the NP was initially located is in this case the unique parameter defining the trench depth. Another situation is encountered when the active NP crosses a step or an edge of a second superimposed FLG sheet, the case of a step-up configuration. In this situation, the height of the trench changes, as the NP remains in contact with the initial basal plane. This feature has been identified for the first time by the actual study within the nanometric resolution of electron tomography in the z direction. For illustration, Fig. 4a,b (4b is rotated with 30° in comparison with 4a) display the TEM view of the area chosen for the tomographic analysis and a longitudinal slice through the reconstructed volume. This slice has been taken in the close vicinity of a long trench traversing several regions with different heights defined by the steps. No change in the cutting direction has been identified even though the NP contacts a step with a height smaller than its size, only channel depth changes, as displayed in Fig. 4c . Indeed, the trench profile varies when the NP crosses areas with different thicknesses. If one takes into account the relation between trenches profile and the NPs shape (see Fig. 3b ), one observes that the trenches geometry correspond exactly to the geometrical characteristics of the NP at the origin of the trench ( Fig. 4c ). This correlation confirms that even on the non-flat areas (that is, step-like surfaces), the NPs remain in contact with the initial basal plane during the entire cutting process and the section of the active NP is a function of the step-up height. In the work of Severin et al . [20] this effect is also shown by means of atomic force microscopy. The original points highlighted by Fig. 4 concern the ability of the electron tomography to provide primary visual 3D information on the shape of the trenches, with the emphasis on the walls characteristics. The depth and width of the as-created trench will continuously change along its length, as they are imposed by the evolution of the cutting thickness within the FLG support. It is evident that these changes are closely imposed and controlled by the initial etching plane and the corresponding diameter of the active NP at given depths along the trench length. 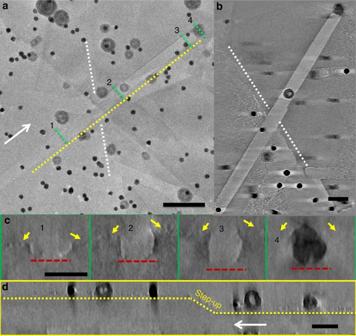Figure 4: The impact of a step-up topographic event on the cutting process. (a) TEM projection of a selected trench and the corresponding NP (scale bar, 50 nm). (b) XY slice through the reconstructed volume of the area shown inFig. 4a(scale bar, 20 nm). The white dotted lines mark the edge of the step-up and the white arrow indicates the cutting direction. (c) XZ slices through the selected trench taken on the numbered positions indicated inFig. 4a(scale bar, 10 nm). The yellow arrows point to the upper FLG surface, whereas the red dotted lines show the trench bottom surface. (d) YZ slice redrawn from a region close to one of the trench wall as marked by the yellow dotted line inFig. 4a(scale bar, 20 nm). Figure 4: The impact of a step-up topographic event on the cutting process. ( a ) TEM projection of a selected trench and the corresponding NP (scale bar, 50 nm). ( b ) XY slice through the reconstructed volume of the area shown in Fig. 4a (scale bar, 20 nm). The white dotted lines mark the edge of the step-up and the white arrow indicates the cutting direction. ( c ) XZ slices through the selected trench taken on the numbered positions indicated in Fig. 4a (scale bar, 10 nm). The yellow arrows point to the upper FLG surface, whereas the red dotted lines show the trench bottom surface. ( d ) YZ slice redrawn from a region close to one of the trench wall as marked by the yellow dotted line in Fig. 4a (scale bar, 20 nm). Full size image A completely different situation is observed when the active NPs cross steps with heights higher than their diameters. In this case, one would expect the NPs to create subsurface cutting, that is, tunnels, according to Lukas et al . [23] Indeed, our 3D analysis allows a direct visualization of these tunnels developing inside the FLG, as evidenced by a series of TEM tomography slices presented in Fig. 5 . According to the cross-sectional slices redrawn from the volume ( Fig. 5c,d ), one can state that we deal with tunnels dug by the iron-based NPs that came in contact with the steps thicker than the NP diameter. Moreover, the slices displayed in Fig. 5c,d show that even under these conditions, the basal plane of the active NPs remains unchanged. 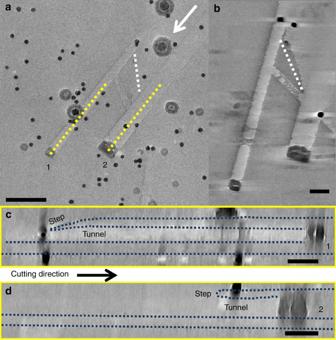Figure 5: Tunnel formation within the FLG support. (a) TEM projection of two selected trenches (scale bar, 50 nm). (b) XY slice extracted from the reconstructed volume of the region presented inFig. 5a(scale bar, 20 nm). The white dotted line indicating the position of the step-up and the white arrow points the cutting direction. (c,d) YZ slices redrawn from the reconstructed volume along the direction marked by the yellow lines inFig. 5a(scale bar, 20 nm). The exact position of the FLG limiting planes is highlighted by blue dot line. Figure 5: Tunnel formation within the FLG support. ( a ) TEM projection of two selected trenches (scale bar, 50 nm). ( b ) XY slice extracted from the reconstructed volume of the region presented in Fig. 5a (scale bar, 20 nm). The white dotted line indicating the position of the step-up and the white arrow points the cutting direction. ( c , d ) YZ slices redrawn from the reconstructed volume along the direction marked by the yellow lines in Fig. 5a (scale bar, 20 nm). The exact position of the FLG limiting planes is highlighted by blue dot line. Full size image When the active NPs cross a step-down defined as a topographical feature on the FLG surface, another trench or an FLG-free edge ( Fig. 6 ), the cutting process can either stop or the cutting direction changes. This ‘free edge sensitivity’ behaviour can be attributed to the adhesion between carbon atoms and the NP facets, more specifically the contact area between the NP facets and the trench walls. This strongly depends on the NP size, shape and position in the trench. The case presented in Fig. 6a–d corresponds to the stop cutting when the NP encounters the border of another trench. 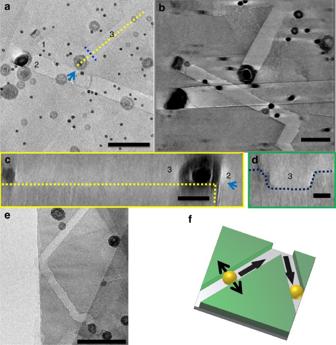Figure 6: The role of a step-down topographic event on the cutting process. (a) TEM projection of a nanostructured area (scale bar, 50 nm) (b) XY slice redrawn from the reconstructed volume (scale bar, 40 nm) displaying the intersection of the trenches 1, 2 and 3 froma. (c) YZ slice taken through the centre of the trench number 3 (scale bar, 20 nm). (d) XZ slice within the volume redrawn from the region marked by the dot blue line in a (scale bar, 10 nm). (e) TEM projection showing the interaction of an active NP with a free FLG edge (scale bar, 50 nm). (f) Schematic representation of the interaction between an NP encountering a FLG edge. Figure 6a,b display 2D TEM images of the selected area and the corresponding longitudinal slice from the reconstructed volume, respectively. Let us design by 1, 2 and 3 several types of trenches defined by different trajectories of the corresponding active NPs and implicitly by different trench topographies. The trench 2 from Fig. 6c appears to be too deep to be crossed by the NP 3 behaviour, which can be attributed to the lack of the frontal adhesion force as the primary source for the NP motion. In the case of the trench 3, the carbon walls are almost identical in terms of height. Two causes can be assigned to ending of the cutting process: the lateral forces acting in opposite directions at the interface NP/carbon walls (see Fig. 6f ) and the blockade created by the trench geometry. A different situation is displayed in Fig. 6e , when the NP is changing direction while approaching the margin of the FLG with a sharp incidence angle between the cutting direction and the FLG-free edge. We attribute this to the disequilibrium of the lateral forces acting between the NP facets/carbon walls. Thereby resuming, there are several parameters controlling the cutting behaviour of an NP approaching free FLG edges: the contact area between NP facets and the trench walls, the incidence angle, the NP size, shape and the trench depth. Although this phenomenon has already been described [16] , [17] , [18] , [29] , the electron tomography as the main approach is reported herein for the first time. Figure 6: The role of a step-down topographic event on the cutting process. ( a ) TEM projection of a nanostructured area (scale bar, 50 nm) ( b ) XY slice redrawn from the reconstructed volume (scale bar, 40 nm) displaying the intersection of the trenches 1, 2 and 3 from a . ( c ) YZ slice taken through the centre of the trench number 3 (scale bar, 20 nm). ( d ) XZ slice within the volume redrawn from the region marked by the dot blue line in a (scale bar, 10 nm). ( e ) TEM projection showing the interaction of an active NP with a free FLG edge (scale bar, 50 nm). ( f ) Schematic representation of the interaction between an NP encountering a FLG edge. Full size image A last important output of this electron tomography-based investigation concerns the core-shell NPs. One deals with two types of core-shell NPs: NPs marked by a hollow between the core and the shell and NPs showing simple hollow characterized by a cavity connecting the outer side with the core cavity (see Supplementary Fig. 4 ). The first conclusion redrawn from the results shown above relies on the complexity of the process of catalytic cutting of the FLG sheets. It strongly depends on both the topography of the carbon support and the morphology of the active catalyst. One first finding relates to the higher activity of the metallic iron as compared with the iron oxide. From a morphological point of view, two types of NPs are distinguished, with homogeneous and hollow morphologies. An explanation for such complex internal structure for the hollow NPs can be searched by referring to the Kirkendall reduction mechanism [30] . Accordingly, the formation of a void in contact with a substrate is governed by the diffusion of chemical species along the crystallographic defects within the NPs. We have shown that the initial deposition of Fe 3− x O 4 NPs on both sides of the FLG sheets induces a dual side cutting. This demonstrates the capacity of the catalytic hydrogenation to improve the bulk properties of FLG by generating a porous network with high accessibility. Owing to the difficulties encountered during a 3D analysis, up to now, no valuable proof has been provided to precisely locate the trenches within the FLG support. Based on 2D imaging only, the hypothesis advanced in a first approach was that we deal with the presence of intersecting trenches with different depths, located most probably on the same side of the FLG support. Owing to its ability to furnish a 3D overview, the electron tomography identified the presence of independent non-intersecting trenches with different depths on both sides of the FLG support. One therefore associates the different contrasts in the 2D micrographs to the superposition effects rather than to the intersecting trenches. The active NPs are generally located at the edges of FLG sheets or attached to the steps on planar surfaces, with no significant cutting activity for the latters. As the 3D character of the active NP is the main factor imposing the trench profile (the walls shape), it is clear that for creating straight nanopatterns with smooth walls, a sharp control of active NP shape is imperative. In this context, further investigations are necessary on one hand for adjusting the shape of the active NPs and to refine the selectivity of the deposited NPs on the edges and steps, on the other hand. The motion of the active NP during cutting is defined by the basal graphitic planes on which the NP fixes initially. The basal plane and the cutting direction do not change even when the NP crosses obstacles with ‘step-up’ configurations defined by topographical steps or superimposed FLG sheets. If the thickness of these step-up obstacles exceeds the size of the NP, one assists at the creation of sub-surface channels (tunnels). By using the electron tomography as the main tool, the formation of tunnels as previously described by Lukas et al . [23] is directly confirmed. Nevertheless, the mechanisms responsible for this rather unexpected behaviour remain unclear. The mechanism of tunnel formation relates to the mechanism of H 2 supply on the active side of the NP, that is, the front side and the CH 4 elimination. Although the proposed diffusion through the graphene layers can partially explain the H 2 supply, it is uncertain that the same paths (saturated with H 2 ) can serve for the elimination of a larger molecule as CH 4 . When the active NP meets a ‘step-down’ event, more precisely a pre-existing topographical feature on the surface, or another trench previously created, one assists at cutting stop or a change of the cutting direction. Sample preparation The FLG sheets have been synthesized by mechanical ablation of pencil leads assisted by an ultrasonication process and followed by acid/base purification to remove the inorganic binder and separation from the weakly ablated species by decantation in toluene [24] , [25] . The decoration of the FLG surface by homogeneous Fe 3− x O 4 NPs was carried out using a solvothermal synthesis [26] , [27] consisting in the thermal decomposition of iron stearate complex in a high boiling solvent, and in the presence of oleic acid (as surfactant) and the FLG. In the solvothermal synthesis, 300 mg of FLG were dispersed in 20 ml of octyl ether (Alfa Aesar, 99%) under ultrasonication for 30 min. After addition of 1.382 g (2.2 mmol) of iron stearate (Fe-stereate Strem Chemicals, (9–10% Fe)) and 1.4 ml (4.4 mmol) of oleic acid (Alfa Aesar, 99%), the whole environment was heated up to 110 °C without cooling. The goal of this latter operation was to dissolve the reactants and to eliminate the water and/or impurities. The cooling condenser has been then added and the system was heated up to reflux (~290 °C) under air, with a heating rate of 5 °C min −1 . The reaction mixture was then kept for 2 h at this temperature. After cooling, the NPs and FLG are precipitated by adding an excess of acetone, followed by a centrifugation with 8,000 r.p.m. for 10 min. The resulting black precipitate was washed three times by hexane:acetone mixture (50:50) and centrifuged (8,000 r.p.m., 10 min). The cutting of FLG by catalytic hydrogenation was performed ex-situ in a tubular reactor at 800 °C with a heating rate of 1,600 °C h −1 under H 2 (total flow rate of 300 ml min −1 ). The cutting (etching) experiment was carried out for 2 h and the sample was then recovered for TEM analysis. TEM, HR-TEM and STEM–EELS investigations For the TEM analyses, a drop of solution containing the etched FLG/NPs aggregates was deposited on a TEM grid covered by a holey carbon membrane. Conventional and HR-TEM images were recorded on a JEOL 2100F microscope working at 200 kV, equipped with a Cs probe corrector and a GATAN Tridiem imaging filter. Spatial-resolved EELS measurements, as well as HR–STEM studies were performed on probe-corrected STEM FEI Titan Low-Base 60–300 operating at 120 kV (fitted with an X-FEG gun and Cs-probe corrector (CESCOR from CEOS GmbH)). EEL spectra were recorded using the spectrum-imaging mode [31] , [32] in a Gatan GIF Tridiem ESR spectrometer. The convergent and the collection semi-angles used for the data acquisition were 25 and 80 mrad, respectively, whereas the energy resolution was ~1.2 eV. Electron tomography The tomography series were obtained for tilting angles from −65° to +65° with a 2° Saxton scheme and subsequent series alignments were performed in the IMOD [33] software using 5-nm gold NPs as fiducial markers. Two types of reconstruction algorithms were used: a SIRT and a DART. For resolving the in-depth details at maximum resolution, we used the SIRT algorithm implemented in a fast software running on multicore computers, Tomo3D [34] . The size of the TEM projections used for the reconstruction was 2k × 2k pixels and the tomogram thickness has been fixed at 2k. Owing to the low contrast of the FLG, to obtain the large-scale segmentation of the tomograms is not trivial. Therefore, we have used the segmentation abilities given by the discrete tomographic algorithms. To get suitable grey values of both the FLG and NPs for further segmentation, a masked SIRT step has been performed by following the steps described by Zuerner et al . [35] The unmasked SIRT reconstruction was analysed to find the most probable boundaries within the layer. Using the masked SIRT reconstruction as a starting model and taking the grey values of its histogram as basis, the DART step was performed. It is important to specify that the DART has been employed to improve data segmentation and subsequent modelling, whereas the volume analysis has been carried out on the volume reconstructed using the SIRT algorithm. How to cite this article: Melinte, G. et al . A 3D insight on the catalytic nanostructuration of few-layer graphene. Nat. Commun. 5:4109 doi: 10.1038/ncomms5109 (2014).